CARMIL leading edge localization depends on a non-canonical PH domain and dimerization CARMIL is an approximately 1,370-amino-acid cytoskeletal scaffold that has crucial roles in cell motility and tissue development through interactions with cytoskeletal effectors and regulation of capping protein at the leading edge. However, the mechanism of CARMIL leading edge localization is unknown. Here we show that CARMIL interacts directly with the plasma membrane through its amino-terminal region. The crystal structure of CARMIL 1–668 reveals that this region harbours a non-canonical pleckstrin homology (PH) domain connected to a 16-leucine-rich repeat domain. Lipid binding is mediated by the PH domain, but is further enhanced by a central helical domain. Small-angle X-ray scattering reveals that the helical domain mediates antiparallel dimerization, properly positioning the PH domains for simultaneous membrane interaction. In cells, deletion of the PH domain impairs leading edge localization. The results support a direct membrane-binding mechanism for CARMIL localization at the leading edge, where it regulates cytoskeletal effectors and motility. Actin-based cell motility underlies many fundamental biological processes, such as dendritic spine formation, immune response and tumour metastasis [1] , [2] , [3] . During these processes, actin filaments form highly dynamic networks at the leading edge of motile cells, with their fast-growing barbed (or +) ends directed towards the plasma membrane (PM), providing the forces for cell motility [4] . As a consequence, actin barbed-end polymerization is tightly regulated in cells via membrane-associated proteins. An important and ubiquitous regulator of barbed-end dynamics is capping protein (CP) [5] . CP binds tightly to the barbed end, which prevents actin monomer addition or dissociation [6] . In this way, CP promotes the formation of actin networks consisting of shorter and more densely branched filaments, thought to be necessary for efficient lamellipodial protrusion [4] , [7] . CP is one of a small subset of cytoskeletal proteins required for reconstitution of actin-based motility in vitro [8] , and is a crucial component of the dendritic actin polymerization model [4] . Despite its critical role in the regulation of actin dynamics, CP lacks a mechanism for direct membrane association and is itself regulated by multiple proteins that could provide a link to the membrane [5] , [7] . The proteins that regulate CP, including CARMIL (CP Arp2/3 complex myosin-I linker), CD2AP, CKIP-1, CapZIP and FAM21, are generally unrelated, but most use a similar allosteric mechanism; they contain a conserved ~30-aa CP interaction (CPI) motif that binds to CP on the opposite side from the actin filament, lowering its affinity for the barbed end [9] , [10] . CARMIL contains, in addition to the CPI motif, a ~14-aa so-called CARMIL-specific interaction motif that also participates in interaction with CP [10] . CARMIL is a large (~1,370-aa) multi-domain protein originally identified as a binding partner of the SH3 domain of myosin-I (refs 11 , 12 , 13 , 14 ). The interaction with myosin-I has been mapped to the carboxy-terminal proline-rich domain (PRD) of CARMIL [12] , which features six canonical SH3-binding PxxP sites ( Fig. 1a ). Vertebrates express three CARMIL isoforms (CARMIL1–3) that have non-overlapping roles in cell motility [15] . CARMIL3 is an oncofetal protein, whose overexpression promotes cell proliferation and tumour growth in adult mice [16] . CARMIL2, which is downregulated in patients affected by psoriasis [17] , colocalizes with the vimentin filament network, and loss of its function impairs cell polarity and motility [15] . CARMIL1 (referred to here simply as CARMIL) has been more extensively studied; it colocalizes with CP at the cell leading edge and its knockdown results in loss of lamellipodial actin and strong inhibition of cell motility and macropinocytosis [15] , [18] . In neuronal cells, CARMIL negatively regulates Trio (UNC-73), a Rho-family GTPase guanine nucleotide exchange factor [19] , resulting in inhibition of axon growth cone migration [15] , [20] . Because of its role in the regulation of actin dynamics, CARMIL is considered a key factor in normal cell motility and tissue development, as well as in aberrant migration of metastatic cancer cells [7] . Yet, with the exception of its interaction with CP [10] , [21] , [22] , [23] , [24] , [25] , the structural and biochemical properties of this large cytoskeletal effector and its mechanism of leading edge localization are poorly understood. 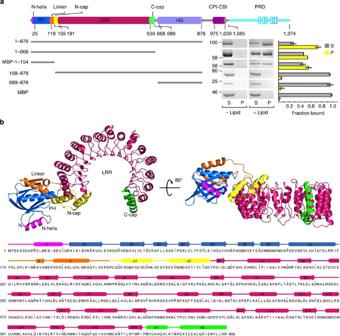Figure 1: Identification of a lipid-binding domain and structure of CARMIL1–668. (a) Domain organization of CARMIL, design of protein constructs and sedimentation with brain lipid extracts. CARMIL was known to contain an LRR domain, although its size and boundaries were unknown, a CPI–CARMIL-specific interaction (CSI) motif and a PRD. Here, through sequence and structural analyses, we have defined the exact boundaries of the LRR domain and identified previously unknown N- and C-terminal caps of the LRR, and two additional domains, a PH domain and a HD. The PH domain is interconnected with an N-terminal helix (N-helix) and a C-terminal linker (Linker). CARMIL constructs (5 μM) were tested for their ability to cosediment with brain lipid extracts (1 mg ml−1). MBP was used as a control. Proteins were centrifuged in the absence or presence of lipids. Positions of molecular weight markers are indicated. Coomassie-stained gel bands were quantified. Error bars represent s.d. from three independent experiments. (b) Two perpendicular representations of the crystal structure of CARMIL1–668, with domains coloured as ina. A representation of the secondary structure and domain assignments resulting from the structure is shown above the sequence of CARMIL1–668, coloured according toa. Figure 1: Identification of a lipid-binding domain and structure of CARMIL 1–668 . ( a ) Domain organization of CARMIL, design of protein constructs and sedimentation with brain lipid extracts. CARMIL was known to contain an LRR domain, although its size and boundaries were unknown, a CPI–CARMIL-specific interaction (CSI) motif and a PRD. Here, through sequence and structural analyses, we have defined the exact boundaries of the LRR domain and identified previously unknown N- and C-terminal caps of the LRR, and two additional domains, a PH domain and a HD. The PH domain is interconnected with an N-terminal helix (N-helix) and a C-terminal linker (Linker). CARMIL constructs (5 μM) were tested for their ability to cosediment with brain lipid extracts (1 mg ml −1 ). MBP was used as a control. Proteins were centrifuged in the absence or presence of lipids. Positions of molecular weight markers are indicated. Coomassie-stained gel bands were quantified. Error bars represent s.d. from three independent experiments. ( b ) Two perpendicular representations of the crystal structure of CARMIL 1–668 , with domains coloured as in a . A representation of the secondary structure and domain assignments resulting from the structure is shown above the sequence of CARMIL 1–668 , coloured according to a . Full size image Here we advance our understanding of CARMIL structure–function by identifying two previously unknown domains: a pleckstrin homology (PH) domain implicated in direct interaction with the PM, and a central helical domain (HD) that mediates antiparallel dimerization and enhances membrane binding by positioning the PH domains for optimal interaction with the membrane. Cellular studies confirm the role of the PH domain in leading edge localization. When combined, the results lead to a new model of CARMIL localization and function at the leading edge. CARMIL binds lipid membranes through its amino-terminal region We sought to determine the mechanism by which CARMIL localizes to the PM in a CP-independent manner [15] , [18] . Prior studies had identified three domains in CARMIL: the leucine-rich repeat (LRR) domain, whose exact boundaries remained unclear, the CPI–CARMIL-specific interaction motif and the carboxy-terminal PRD. Through sequence analysis, we identified what appeared to be two additional domains, a ~150-aa N-terminal domain clearly distinguished from the LRR domain by its predicted high β-strand content, and a predicted HD (residues 689–878 of mouse CARMIL1, the species studied here) positioned between the LRR and CPI domains ( Fig. 1a ). We expressed fragments corresponding to each of these individual domains as well as combinations of domains ( Fig. 1a ). CARMIL 1–154 had limited solubility on its own, and was expressed as a maltose-binding protein (MBP) fusion, which increased its solubility. To test whether CARMIL could directly bind lipid membranes, we assessed the ability of each construct to cosediment with liposomes derived from bovine brain lipid extracts (Folch fraction I). In the absence of lipids, all the constructs were soluble and did not sediment ( Fig. 1a and Supplementary Fig. S1 ). In the presence of lipids, constructs containing the N-terminal domain cosedimented with lipids ( Fig. 1a ). Interestingly, CARMIL 1–878 , including the HD, cosedimented more abundantly than MBP-CARMIL 1–154 and CARMIL 1–668 (80% versus 55%). This was a surprising result, as the isolated HD, CARMIL 689–878 , did not cosediment with lipids. When combined, these findings suggested that the N-terminal region of CARMIL directly binds lipid membranes, whereas the HD contributes indirectly to this activity (addressed below). Crystal structure of CARMIL 1–668 The N-terminal domain of CARMIL implicated above in lipid binding had no detectable sequence similarity with any known structure. Therefore, to understand the molecular basis for lipid binding, we sought to determine its structure. Multiple N-terminal fragments were expressed, but they all had poor solubility. The isolated LRR domain also had low solubility. In contrast, CARMIL 1–668 , comprising the N-terminal and LRR domains, was highly soluble, suggesting that these two domains were structurally interconnected. CARMIL 1–668 was crystallized and its structure was determined using the single-wavelength anomalous dispersion method ( Fig. 1b , Table 1 , Supplementary Fig. S2 and Supplementary Movie 1 ). The structure was refined to 2.9 Å resolution using four-fold non-crystallographic symmetry constraints, and revealed two major domains: a PH domain (residues 25–118) and a 16-LRR domain (residues 191–638). Table 1 Data collection and refinement. Full size table The PH domain is a recognized lipid-binding fold [26] , which is consistent with the ability of the N-terminal region of CARMIL to cosediment with lipid extracts. It is not surprising, however, that the PH domain of CARMIL had remained undetected from sequence, as it displays multiple non-canonical features. The most closely related canonical PH domains identified with the programme Dali [27] share ≤12% sequence identity with that of CARMIL ( Supplementary Fig. S3 ). The PH domain fold consists of a seven-strand β-barrel, capped at one end by a C-terminal α-helix, whereas the other end of the β-barrel hosts the lipid-binding pocket [28] . Although these features are conserved in the PH domain of CARMIL, key residues in the lipid-binding pocket are not conserved ( Supplementary Fig. S3 ). Moreover, the PH domain of CARMIL is tightly integrated with N- and C-terminal structural elements that do not form part of the canonical PH fold. These include an α-helix at the N terminus (residues 10–20), referred to here as the N-helix, and a β-strand followed by an α-helix at the C terminus (residues 129–147), referred to here as the Linker region ( Fig. 1b and Supplementary Fig. S2b ). The β-strand in the Linker region is incorporated as an additional strand into the β-barrel of the PH domain. The Linker region is conserved within each CARMIL isoform, but not across isoforms ( Supplementary Fig. S4 ), suggesting that it might perform isoform-specific functions in addition to linking the PH and LRR domains. The LRR domain has an overall planar horseshoe shape with an inner radius ( r ) of ~19 Å and spans an arc angle ( ϕ ) of ~232° ( Supplementary Fig. S5a ) [29] . The LRR domain of CARMIL is most closely related to that of ribonuclease inhibitor [30] , but has a somewhat more elliptical shape. Each LRR motif consists of a β-strand, occupying the inner side of the LRR domain, and an α-helix on the outer side of the domain. The loop connecting these two secondary structure elements is called the ‘ascending loop’, whereas that connecting one repeat to the next is called the ‘descending loop’. In CARMIL, only repeat 6 displays a fully canonical LRR sequence (LxxLxLxxN/CxL) ( Supplementary Fig. S5b ) and was thus used as a reference in comparisons with the other repeats. Repeats 3–15 overlay well with repeat 6, with an average root-mean-square displacement (RMSD) for equivalent Cα-atoms of 0.65 Å, whereas repeats 1, 2 and the incomplete repeat 16 diverge more significantly ( Supplementary Fig. S5c ). The LRR of CARMIL is capped at the N- and C-terminal ends by helix-loop-helix motifs. These caps are highly conserved among CARMIL isoforms, particularly the N-terminal cap ( Supplementary Fig. S4 ). Both caps contain a helix that runs diagonally to the first (or the last) LRR motif, such that it shields the hydrophobic core of the LRR domain from solvent exposure ( Supplementary Fig. S5d,e ). Although such caps are common among LRR-containing proteins and are thought to stabilize their structures [29] , those of CARMIL are distinct from other known LRR capping motifs. Only one other protein, tropomodulin [31] , contains a helix within its C-terminal cap that superimposes well with that of CARMIL ( Supplementary Fig. S5f ). The PH domain and lipid binding PH domains are often implicated in phospholipid binding [26] . Therefore, we asked whether the PH domain of CARMIL bound specific phospholipids, accounting for the cosedimentation observed with brain lipid membranes ( Fig. 1a ). Using a lipid strip assay [32] , we found that CARMIL 1–878 , the fragment that cosedimented most abundantly with lipid membranes, showed specificity for phosphatidylinositol, phosphatidylserine (PS) and monophosphorylated phosphatidylinositides (PtdIns(3)P, PtdIns(4)P and PtdIns(5)P) ( Fig. 2a ). However, contrary to most canonical PH domains, CARMIL 1–878 did not appear to bind polyphosphorylated phosphatidylinositides. PS accounts for ~12% of the lipid content of the inner leaflet of the PM [33] , suggesting that CARMIL could bind directly to the PM through its PH domain. Accordingly, CARMIL 158–878 , in which the PH domain was deleted, showed no lipid-binding activity ( Fig. 2a ), which is consistent with the inability of this fragment to cosediment with lipid membranes ( Fig. 1a ). 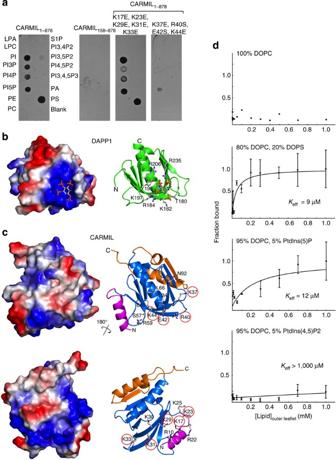Figure 2: Specificity and affinity of lipid binding. (a) Lipid-binding specificity of CARMIL constructs and PH domain mutants (60 nM) using a lipid overlay assay (Echelon Biosciences). Each experiment was repeated three times. (b) Surface charge distribution and cartoon representation of the canonical PH domain of DAPP1 with bound PtdIns(1,3,4,5)P4 (PDB ID: 1FAO), used as reference for comparison with the PH domain of CARMIL. Residues important for ligand binding are shown. (c) Two views of the PH domain of CARMIL, including the N-helix (magenta) and Linker (orange), which form a structural unit with the PH domain. The top view is the same as for DAPP1 and highlights differences in the canonical lipid-binding pocket. The bottom view shows a highly basic pocket formed at the interface between the PH domain and the N-helix. Residues of both pockets mutated inaare circled. (d) Binding of CARMIL1–878to large unilamellar vesicle (LUVs) with the indicated lipid composition. The fraction of CARMIL1–878(5 μM) cosedimenting with LUVs is plotted as a function of outer leaflet lipid concentration. Error bars represent s.d. from three independent experiments. Solid lines represent the best fit of the data. Effective lipid-binding affinities are indicated. Figure 2: Specificity and affinity of lipid binding. ( a ) Lipid-binding specificity of CARMIL constructs and PH domain mutants (60 nM) using a lipid overlay assay (Echelon Biosciences). Each experiment was repeated three times. ( b ) Surface charge distribution and cartoon representation of the canonical PH domain of DAPP1 with bound PtdIns(1,3,4,5)P4 (PDB ID: 1FAO), used as reference for comparison with the PH domain of CARMIL. Residues important for ligand binding are shown. ( c ) Two views of the PH domain of CARMIL, including the N-helix (magenta) and Linker (orange), which form a structural unit with the PH domain. The top view is the same as for DAPP1 and highlights differences in the canonical lipid-binding pocket. The bottom view shows a highly basic pocket formed at the interface between the PH domain and the N-helix. Residues of both pockets mutated in a are circled. ( d ) Binding of CARMIL 1–878 to large unilamellar vesicle (LUVs) with the indicated lipid composition. The fraction of CARMIL 1–878 (5 μM) cosedimenting with LUVs is plotted as a function of outer leaflet lipid concentration. Error bars represent s.d. from three independent experiments. Solid lines represent the best fit of the data. Effective lipid-binding affinities are indicated. Full size image Most PH domains that bind phospholipids with high affinity tend to have conserved residues that form a lipid-binding pocket on one side of the β-barrel and display an overall basic charge around the lipid-binding pocket [26] , [28] . Such is the case of DAPP1, a canonical PH domain identified by Dali [27] as one of the closest structural relatives of CARMIL’s PH domain ( Supplementary Fig. S3 ), which was crystallized with bound PtdIns(1,3,4,5)P4 (ref. 28 and Fig. 2b ). In contrast, the PH domain of CARMIL lacks most of these residues ( Fig. 2c ). However, on the opposite side of the PH domain, at the interface between the N-helix and the PH domain, CARMIL has a prominent basic pocket formed by residues R10, K17, R22, K23, K25, K29, K30, K31 and K33 ( Fig. 2c ). As some PH domains bind lipids through sites other than the classical pocket [34] , we suspected that this pocket in CARMIL could harbour a lipid-binding site. However, a CARMIL 1–878 mutant in which five of these residues (K17, K23, K29, K31 and K33) were all substituted by glutamic acid bound lipids similarly to the wild-type protein in the lipid strip assay ( Fig. 2a ). As this basic pocket had no apparent role in lipid binding, we tested whether the canonical lipid-binding pocket was functional. Three basic residues surround this pocket in CARMIL (K37, R40 and K44). A CARMIL 1–878 mutant in which these three residues were replaced by glutamic acid, and E42 in the middle of the pocket was substituted by serine, did not bind lipids in the strip assay. We thus conclude that despite its unusual properties the lipid-binding pocket in the PH domain of CARMIL is still functional, but contrary to most PH domains it appears to have specificity for PS and monophosphorylated lipids. To quantitatively test this possibility, we measured the affinity of CARMIL 1–878 for different types of lipids using a cosedimentation assay ( Fig. 2d ). This assay quantifies the amount of CARMIL 1–878 cosedimenting with large unilamellar vesicles containing lipids identified in the strip assay [35] . Consistent with the strip assays, CARMIL 1–878 did not bind phosphatidylcholine, cosedimented very weakly with PtdIns(4,5)P2, but bound DOPS (1,2-dioleoyl-sn-glycero-3-phospho- L -serine) and PtdIns(5)P with ~10 μM affinity. These results suggest that membrane binding by the PH domain of CARMIL might be dominated by binding to PS, which is highly abundant in the PM. A central HD mediates antiparallel dimerization CARMIL 1–878 cosedimented ~25% more abundantly with brain lipids than CARMIL 1–668 . These two fragments differ only in that CARMIL 1–878 includes the predicted HD, which had no lipid-binding activity on its own ( Fig. 1a ). Consistent with the secondary structure prediction ( Supplementary Fig. S4 ), the circular dichroism spectrum of CARMIL 689–878 displayed minima at 208 and 222 nm, characteristic of an all-helical structure ( Fig. 3a ). Analysis of CARMIL constructs by size exclusion chromatography (SEC) showed that fragments containing the HD eluted with molecular weight characteristics of dimers, whereas fragments lacking the HD were monomeric ( Fig. 3b and Table 2 ). Note that each mass measurement was carried out with at least two different methods, to account for uncertainties in the mass estimates of elongated proteins derived from SEC ( Table 2 ). At higher concentrations the isolated HD showed limited solubility, but a fusion protein with MBP (MBP-CARMIL 689–878 ) was highly soluble. MBP-CARMIL 689–878 formed a dimer in solution, as determined by analytical SEC and multi-angle light scattering (SEC–MALS), whereas MBP alone was monomeric ( Fig. 3b,c and Table 2 ). These results confirmed that the HD was sufficient for dimerization. 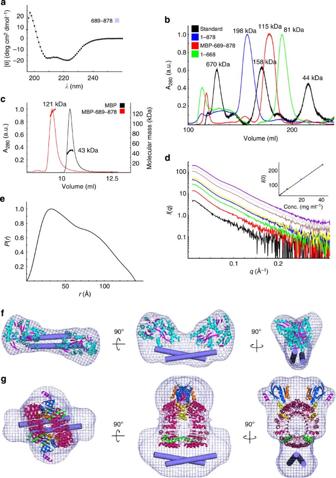Figure 3: CARMIL dimerization. (a) The circular dichroism spectrum of CARMIL689–878displays minima at 208 and 222 nm, characteristic of all-helical structures. (b) Molecular mass estimates from gel filtration. (c) Measurement of the masses of MBP and MBP-CARMIL689–878by SEC–MALS. (d) SAXS intensity plotted versus momentum transfer for different MBP-CARMIL689–878concentrations (1, 2.5, 5, 7.5, 10, 20, 30 and 40 mg ml−1). The I(0) versus concentration plot shown in the inset is linear, demonstrating lack of protein aggregation. (e) Normalized distance distribution function of MBP-CARMIL689–878. (f) Three perpendicular views of the average SAXS envelope of MBP-CARMIL689–878fit with two molecules of MBP (PDB ID: 3Q25). The dimeric HD, whose structure is unknown, is schematically represented by two crossing cylinders (purple). (g) Three perpendicular views of the average SAXS envelope of CARMIL1–878fit with two copies of the structure of CARMIL1–668and a schematic representation of the HD. Figure 3: CARMIL dimerization. ( a ) The circular dichroism spectrum of CARMIL 689–878 displays minima at 208 and 222 nm, characteristic of all-helical structures. ( b ) Molecular mass estimates from gel filtration. ( c ) Measurement of the masses of MBP and MBP-CARMIL 689–878 by SEC–MALS. ( d ) SAXS intensity plotted versus momentum transfer for different MBP-CARMIL 689–878 concentrations (1, 2.5, 5, 7.5, 10, 20, 30 and 40 mg ml −1 ). The I(0) versus concentration plot shown in the inset is linear, demonstrating lack of protein aggregation. ( e ) Normalized distance distribution function of MBP-CARMIL 689–878 . ( f ) Three perpendicular views of the average SAXS envelope of MBP-CARMIL 689–878 fit with two molecules of MBP (PDB ID: 3Q25). The dimeric HD, whose structure is unknown, is schematically represented by two crossing cylinders (purple). ( g ) Three perpendicular views of the average SAXS envelope of CARMIL 1–878 fit with two copies of the structure of CARMIL 1–668 and a schematic representation of the HD. Full size image Table 2 Molecular masses (kDa) estimated by different methods. Full size table To investigate the mechanism of dimerization, we used small-angle X-ray scattering (SAXS). Data collected at several concentrations of MBP-CARMIL 689–878 showed a linear dependence of the scattering intensity with protein concentration ( Fig. 3d ), confirming that this construct does not aggregate even at high concentrations (up to 40 mg ml −1 ). The molecular mass estimated from the scattering intensity at zero angle, I (0), and using glucose isomerase as a standard, was 129 kDa (theoretical mass, 61 kDa), corresponding to a dimer in solution ( Table 2 ). The distance distribution plot generated from the scattering data showed a bimodal distribution, indicative of a dumbbell-shaped molecule ( Fig. 3e ). A molecular envelope was obtained by averaging 20 ab initio structures calculated with the programme DAMMIF [36] . As we had established that MBP-CARMIL 689–878 was dimeric, two-fold symmetry constraints were imposed during the calculations, which substantially improves the quality of the envelope [37] . Consistent with the distance distribution plot, the envelope displayed two distal lobes ( Fig. 3f ). These lobes fit well two globular MBP molecules (molecular mass, 40 kDa). The remaining density corresponded to the HD dimer (molecular mass, 42 kDa), which seemed to have a narrow and elongated shape. The MBP molecules were distally disposed in the envelope, suggesting that the HD associates in an antiparallel manner. To determine the mechanism by which the HD enhances lipid binding by the PH domain, we analysed the structure of CARMIL 1–878 by SAXS. At high concentrations, CARMIL 1–878 was prone to aggregation. Therefore, the scattering data was collected at a single concentration, from protein separated by SEC immediately before data collection. The molecular mass of CARMIL 1–878 estimated from the scattering intensity was 226 kDa, consistent with a dimer, whereas that of CARMIL 1–668 was 80 kDa, consistent with a monomer ( Table 2 ). The distance distribution plots for these two fragments had the characteristic shape of elongated globular proteins [37] ( Supplementary Fig. S6a,b ). An ab initio SAXS envelope of CARMIL 1–878 was generated by imposing two-fold symmetry constraints. The crystal structure of CARMIL 1–668 ( Fig. 1b ) was manually fit as a dimer into the envelope, which could only be accomplished in a single orientation ( Fig. 3g and Supplementary Movie 1 ). The remaining unfilled density was assigned to the antiparallel HD and had approximately the same shape and size as determined above from the envelope of MBP-CARMIL 689–878 ( Supplementary Fig. S6c ). In the resulting model of the dimer, the PH domains project out in the same orientation, such that their lipid-binding pockets can simultaneously interact with the PM. The PH domain mediates leading edge localization in cells The ensemble of our in vitro results implicated the PH domain of CARMIL in membrane binding. To test whether this was also its role in cells, we expressed CARMIL FL -GFP or CARMIL Δ PH -GFP (lacking residues 1–157) in B16F1 cells and compared the ability of these two constructs to localize to the leading edge ( Fig. 4 ). The localization of the CARMIL constructs was quantitatively compared with each other and with that of green fluorescent protein (GFP), after normalization against red fluorescence protein (RFP) fluorescence. Quantification of PM localization was carried out using the PM index [38] , which characterizes the localization along the entire leading edge and avoids errors due to volume effects. Both GFP and RFP displayed diffuse localization (PM index=0). The PM indexes of CARMIL FL -GFP and CARMIL Δ PH -GFP were 1.41 and 0.61, respectively ( Fig. 4 ), corresponding to more than a twofold reduction in PM localization due to deletion of the PH domain. This result indicates that in cells the PH domain functions to recruit CARMIL to the leading edge through direct interaction with the membrane. 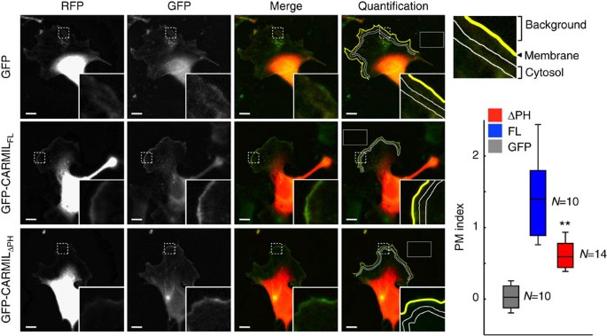Figure 4: Role of the PH domain in leading edge localization of CARMIL. Wide-field fluorescence microscopy of B16F1 cells co-expressing RFP and either GFP, GFP-CARMILFLor GFP-CARMILΔPH(residues 158–1,374). Scale bars, 10 μm. Regions highlighted by dashed boxes are enlarged in insets. Solid boxes indicate areas used to calculate the background fluorescence. The inset shown on the top right corner illustrates the method used to define the background, leading edge and cytosol regions for averaging of fluorescence intensities. Quantifications of the PM index of each construct are given as box-and-whisker plots: box length represents values from low to upper quartile, whiskers encompass 5–95th percentile, boxes are divided by the median. The number of cells analysed for each construct was: GFP, 10; GFP-CARMILFL, 10; and GFP-CARMILΔPH, 14. The statistical significance of the difference between GFP-CARMILFLand GFP-CARMILΔPH, based on the unpaired Student’st-test, is indicated by asterisks (**P<0.01). Figure 4: Role of the PH domain in leading edge localization of CARMIL. Wide-field fluorescence microscopy of B16F1 cells co-expressing RFP and either GFP, GFP-CARMIL FL or GFP-CARMIL ΔPH (residues 158–1,374). Scale bars, 10 μm. Regions highlighted by dashed boxes are enlarged in insets. Solid boxes indicate areas used to calculate the background fluorescence. The inset shown on the top right corner illustrates the method used to define the background, leading edge and cytosol regions for averaging of fluorescence intensities. Quantifications of the PM index of each construct are given as box-and-whisker plots: box length represents values from low to upper quartile, whiskers encompass 5–95th percentile, boxes are divided by the median. The number of cells analysed for each construct was: GFP, 10; GFP-CARMIL FL , 10; and GFP-CARMIL ΔPH , 14. The statistical significance of the difference between GFP-CARMIL FL and GFP-CARMIL ΔPH , based on the unpaired Student’s t -test, is indicated by asterisks (** P <0.01). Full size image CARMIL is an important factor in normal cell motility and tissue development, as well as aberrant migration of metastatic cancer cells [7] . However, although significant effort has been devoted to understanding the interaction of CARMIL with CP and its effect on barbed-end dynamics [10] , [21] , [22] , [23] , [24] , [25] , the structural and functional properties of the other domains of this large cytoskeletal effector remained poorly understood. This study advances our knowledge of CARMIL function, including the identification and characterization of two previously unknown domains N- and C-terminal to the LRR domain: a PH domain involved in direct binding to the PM and a HD responsible for antiparallel dimerization and enhancement of CARMIL’s membrane-binding activity. The PH domain of CARMIL had remained undetected because of its low sequence identity with canonical PH domains ( Supplementary Fig. S3 ). Structural features also set it apart, including its tight integration with N- and C-terminal structural elements (N-helix and Linker), which are not part of the canonical PH fold, and a lipid-binding pocket with substitutions of most of the conserved residues in canonical PH domains [26] . At the biochemical level, these differences translate into the rather unusual lipid specificity of this PH domain, adapted for interaction with monophosphorylated lipids, particularly PS ( Fig. 2 ). Given the relative abundance of PS at the PM [33] , it appears that CARMIL’s PH domain mediates non-specific binding to the membrane, in contrast to other PH domains that bind polyphosphorylated phosphatidylinositides, which are thought to function as signalling lipids [35] . Signalling lipids exist transiently in the membrane, are spatially segregated and are present in low amounts [39] . In contrast, PS is uniformly distributed, such that the observed enrichment of CARMIL at the leading edge ( Fig. 4 ) must be due in part to interactions with other factors. One such factor could be myosin-I, whose SH3 domain binds to the C-terminal PRD of CARMIL [11] , [12] , [13] , [14] , and which also contains a PH domain that allows it to bind independently to the PM [40] . Another binding partner of CARMIL, Trio [15] , [20] , also contains two PH domains and interacts with GTPases at the membrane through its two guanine-nucleotide exchange factor (GEF) domains [19] . Because of its large modular structure, other binding partners of CARMIL are likely to emerge, offering alternative mechanisms for leading edge localization and regulation of its activity. The PH domain, in particular, is more than a lipid-binding fold, as it frequently becomes involved in protein–protein interactions with membrane-bound partners [41] , enhancing membrane localization by a mechanism known as coincidence detection [42] . Using sedimentation equilibrium, it was previously reported that Acanthamoeba castellanii CARMIL existed in monomer–dimer equilibrium with an association constant of 1.0 × 10 6 M −1 , and it was further suggested that binding to CP promotes CARMIL dimerization to form a 1:2 CP:CARMIL complex [43] . The mammalian isoform studied here appears to function as a constitutive dimer, independent of interaction with CP, as we did not observe any evidence of dissociation. As the binding site for CP is fully contained within a CARMIL monomer [10] , our results also predict that the stoichiometry of the CP:CARMIL complex in cell is 2:2 (one CARMIL dimer to a two CP heterodimers). We further determined the molecular mechanism of dimerization, which is mediated by a ~200-aa central domain that is mostly helical and associates in an antiparallel manner ( Fig. 3 ). These characteristics and the overall dimensions of the HD, which is relatively narrow in two directions and elongated in the third direction, are shared with two other folds that are abundant among cytoskeletal proteins and consist of antiparallel helical bundles, the spectrin repeat and the BAR domain ( Supplementary Fig. S6c ). Through dimerization, all the interactions of CARMIL, including with CP, myosin-I and membranes, are duplicated. In the case of membrane binding, dimerization not only works by duplication of the membrane-binding affinity of the PH domain, as frequently observed with membrane-binding modules [42] , but also by optimally orienting the PH domains such that they can simultaneously bind the membrane ( Fig. 5 ), probably explaining why CARMIL 1–878 cosedimented ~25% more abundantly with membranes than CARMIL 1–668 . 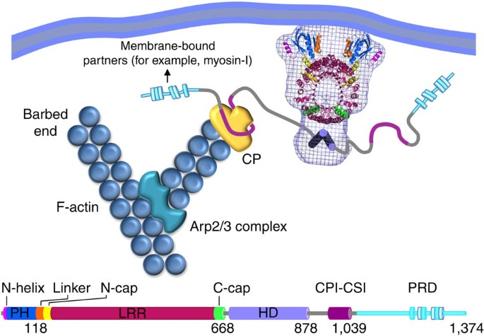Figure 5: CARMIL functional model. CP caps the barbed ends of actin filaments in dendritic networks nucleated by the Arp2/3 complex, resulting in short, densely branched filaments required for cell motility. CARMIL allosterically inhibits the interaction of CP with barbed ends and may also mediate CP’s localization to the leading edge. CARMIL’s own localization to the leading edge likely involves a combination of direct membrane binding by the PH domain, dimerization through the HD and protein–protein interactions with partners such as myosin-I mediated by its other domains. Figure 5: CARMIL functional model. CP caps the barbed ends of actin filaments in dendritic networks nucleated by the Arp2/3 complex, resulting in short, densely branched filaments required for cell motility. CARMIL allosterically inhibits the interaction of CP with barbed ends and may also mediate CP’s localization to the leading edge. CARMIL’s own localization to the leading edge likely involves a combination of direct membrane binding by the PH domain, dimerization through the HD and protein–protein interactions with partners such as myosin-I mediated by its other domains. Full size image Although the HD is sufficient for dimerization, other parts of the CARMIL molecule may participate in dimerization interactions. Indeed, CARMIL 1–668 and CARMIL 1–878 were monomeric and dimeric, respectively, whereas the isolated HD (MBP-CARMIL 689–878 ) was dimeric. Yet, the SAXS envelope of CARMIL 1–878 suggests that the LRR domain may also contribute to the dimerization interface ( Fig. 3g ). Coincidentally, the descending surface of the LRR displays two distinct areas of high sequence conservation at the ends, coinciding with the LRR–LRR contact interface in the dimer ( Supplementary Fig. S2a ). On the other hand, the ascending surface and N-cap regions of the LRR are more uniformly conserved and fully exposed in the dimer, suggesting that these surfaces may be involved in protein–protein interactions, which is the general function of LRR proteins [29] . Large LRR domains typically bind more than one target through different surfaces; CARMIL’s LRR with 16 repeats is also likely to provide a platform for multiple protein–protein interactions. The involvement of CARMIL’s PH domain in membrane localization was demonstrated here in cells, where deletion of the PH domain results in more than a 50% reduction in leading edge localization ( Fig. 4 ). This value probably underestimates the role of the PH domain in membrane localization, as CARMIL Δ PH could have cross-dimerized with endogenous CARMIL in cells, artificially increasing the localization of CARMIL Δ PH at the leading edge. Our results contrast with a previous qualitative analysis, suggesting that a 594-aa N-terminal fragment of CARMIL did not localize to the leading edge [18] . Possible causes for this discrepancy are the inability of this construct to dimerize, a factor shown here to have a key role in leading edge localization, and potential misfolding due to an incomplete LRR domain lacking the C-terminal cap. Whether directly through its PH domain or indirectly through partners, the cellular functions of CARMIL, specifically CARMIL1, are localized at the leading edge of the cell where it controls cell motility [15] , [18] . Interestingly, other CPI-containing proteins are also localized at the membrane, including CD2AP [44] , Fam21 (ref. 45 ) and CKIP-1 (ref. 46 ). In particular, CKIP-1 contains a PH domain, which, similar to that of CARMIL, binds preferentially monophosphorylated lipids and PS [48] . Furthermore, CD2AP, whose leading edge localization depends on interaction with cortactin, was recently shown to recruit CP to the leading edge [46] . It is therefore emerging that proteins that regulate the activity of CP may also regulate its localization at the interface between filament barbed ends and membranes. The ensemble of our results support a model in which the HD and PH domains work synergistically to enhance CARMIL’s localization at the leading edge ( Fig. 5 ), where it interacts with partners such as Trio and myosin-I, and exerts its regulatory function on CP and cell motility. Proteins Mouse CARMIL1 (UniProt ID: Q6EDY6) fragments (see Fig. 1a for details) were cloned into plasmids pMAL-c2E (New England Biolabs) or pRSFDuet-1 (EMD Millipore). The specific primers used for each construct are listed in Supplementary Table S1 . Proteins were expressed in BL21 (DE3)-RIPL cells (Agilent Technologies). Cells were lysed using a Microfluidizer (Microfluidics). Proteins were purified by affinity chromatography (amylose or Ni-NTA resin), followed by additional purification steps through mono-Q and gel filtration columns. Unless otherwise specified, the affinity purification tags (MBP or hexahistidine) were cleaved using TEV protease. Lipid-binding assays Cosedimentation assays with lipids were performed as described [49] , by mixing proteins at 5 μM with 0.6 mg ml −1 brain lipids (Folch fraction I, Sigma), followed by centrifugation at 150,000 g . The supernatant was removed and the pellet was washed with buffer and resuspended. Supernatant and pellet fractions were analysed by SDS–PAGE. The intensities of the bands in the gel were quantified using ImageJ software [50] . Lipid overlay assays were performed using PIP strips (Echelon Biosciences). Membranes were incubated with 60 nM proteins. Proteins were detected with 1,000 × diluted rabbit anti-CARMIL antibodies (Santa Cruz Biotechnology). Membranes were then incubated with anti-rabbit antibody-conjugated horseradish peroxidase (GE Healthcare Life Sciences). Bound CARMIL was then detected using an enhanced chemiluminescence kit (GE Healthcare Life Sciences). Vesicle-binding assays were carried out using large unilamellar vesicles prepared as described [51] . Chloroform-solvated lipids consisting of DOPC (1,2-dioleoyl- sn -glycero-3-phosphocholine) and either 20% DOPS, 5% PtdIns(5)P or 5% brain PtdIns(4,5)P2 (mole fraction) were dried under a nitrogen stream. Note that DOPC and DOPS are commonly used substitutes for naturally occurring PC and PS, which can have varying fatty acid compositions. Lipids were resuspended in 20 mM HEPES pH 7.5 and 176 mM sucrose to a final concentration of 5 mM. Lipid solutions were then subjected to ten cycles of freezing and thawing, bath sonication for 1 min and extrusion through a 100-nm filter using a Mini-Extruder (Avanti Polar Lipids). Lipids were then dialysed in 20 mM HEPES pH 7.5, 200 mM NaCl and 1 mM dithiothreitol (DTT). Vesicle-binding assays were performed as described previously [51] . CARMIL 1–878 at 5 μM was mixed with lipids at various concentrations ranging from 0 to 2 mM and was centrifuged at 150,000 g for 30 min at 20 °C. Supernatant and pellet fractions were analysed by SDS–PAGE and gel band intensities were quantified using ImageJ. Data were fit to a single-site binding equation using Grace software. The apparent affinity constants ( K eff ) were expressed in terms of the total outer membrane lipid concentration. Circular dichroism The far ultraviolet spectrum of CARMIL 689–878 was obtained at a protein concentration of 10 μM in 20 mM phosphate buffer pH 7.5, 200 mM NaCl and 1 mM DTT, using an Aviv Model 410 spectrometer. Measurements were taken at 25 °C. The final normalized circular dichroism spectrum was obtained by subtracting the average of ten buffer-only scans from the average of ten protein scans. SEC and light scattering Samples (10 mg ml −1 ) were fractionated by SEC using a HiLoad 26/60 Superdex 200 column and molecular weights were estimated by comparison with a molecular weight standard (Bio-Rad). For SEC–MALS, samples (5 mg ml −1 ) were separated using a TSK-gel Super SW2000 column (Tosoh Bioscience). Light-scattering measurements were performed using a DAWN HELEOS MALS detector and an Optilab Rex refractive index detector, and molecular masses were estimated using Astra software (Wyatt Technology). Small-angle X-ray scattering Scattering data collection was carried out at the Cornell High Energy Synchrotron Source (CHESS) beamline F2 at 20 °C. CARMIL samples were analysed in 20 mM Tris HCl pH 8.0, 100 mM NaCl, 2 mM DTT. To limit radiation damage, the samples were continuously oscillated inside the cuvette during the 30-s exposures. Six exposures were typically collected from each sample before radiation damage became apparent, as estimated from comparisons of each measurement to the first. Independent measurements were collected from each sample at different concentrations, checking the linear dependence of the scattering intensity at zero angle as a function of concentration to ensure lack of aggregation. One of the samples, CARMIL 1–878 , was prone to aggregation. This sample was pre-concentrated to 12 mg ml −1 and run through a SD200 gel filtration column, and data were collected immediately after elution of the dimeric peak. Data normalization, solvent subtraction and Guinier analysis were done using the BioXTAS RAW software. Data analysis was carried out using the ATSAS software suite, including the programmes GNOM [52] , used to calculate the distance distribution function P ( r ), and DAMMIF [36] , used in automated bead modelling for shape determination. To generate the models of the dimeric samples MBP-CARMIL 689–878 and CARMIL 1–878 , two-fold symmetry constraints were imposed, which produces more reliable envelopes by reducing noise [37] . For each sample, 20 independent shape models calculated with DAMMIF were averaged using DAMAVER [53] to produce the final ab initio envelopes. Crystallography Crystals of CARMIL 1–668 (10 mg ml −1 ) in 20 mM Tris HCl pH 8.0, 100 mM NaCl and 2 mM DTT were obtained at 20 °C in hanging drops containing a 1:0.5:0.5 (v/v) mixture of protein solution, well solution (130 mM Li 2 SO 4 and 16% PEG 3350) and Silver Bullets 71 (Hampton Research). Crystals belonging to space group P1 ( Table 1 ) grew to their final size after 48 h. Crystals of a Se-Met derivative were grown under similar conditions by mixing the protein solution at 30:1 (v/v) ratio with a seeding solution of crushed native crystals in crystallization buffer. For data collection, crystals were flash frozen in liquid nitrogen from a cryosolution consisting of crystallization buffer supplemented with 11% PEG 1,000 and 11% PEG 400. X-ray data collection was carried out at National Synchrotron Light Source beamline X6A. Data were indexed and scaled using HKL2000 (ref. 52 ). Experimental phases were determined using the single-wavelength anomalous dispersion method. SnB [55] was the only programme capable of finding 56 correct solutions out of the 76 selenium atoms expected for the four molecules in the P1 unit cell. The positions of the selenium atoms were refined with the programme Phenix [56] . Phenix also detected the four-fold non-crystallographic symmetry operators, found additional sites, removed six wrong sites and automatically built parts of the structure into the fourfold averaged electron density map. Additional model building was carried out manually, using the programme Coot [55] . The statistics of the final Phenix-refined model are given in Table 1 . Expression and visualization of CARMIL constructs in cells B16F1 mouse melanoma cells were cultured as described [56] . Cells were cotransfected with RFP and either GFP, GFP-CARMIL FL or GFP-CARMIL ΔPH using Lipofectamine LTX and Plus reagents (Invitrogen). Light microscopy was performed using a Nikon Eclipse TE2000U Inverted Microscope equipped with a Planapo 100 × 1.3 numerical aperture objective and a Cascade 512B CCD camera (Photometrics) driven by the MetaMorph imaging software (Molecular Devices). The average fluorescence intensity of a 0.46-μm wide line drawn along the entire leading edge was compared with the intensity in the cytosol, defined as a 3-μm band separated by 3 μm from the leading edge (as depicted in Fig. 4a ). Membrane ruffles were excluded from this analysis. Intensities were measured using ImageJ [50] . The background fluorescence intensity, measured from a rectangle outside the cell, was subtracted from the average intensities of the leading edge and the cytosol. The expression of RFP was used to control for volume fluctuation in the cell. The PM index, a measure of the membrane-bound fraction of each construct, was calculated as described [38] , using the equation: PM index=((GFPm/GFPc)/(RFPm/RFPc))−1, where GFPm, GFPc, RFPm and RFPc are the average fluorescence intensities of GFP and RFP at the leading edge or in the cytosol after subtraction of the background intensity. The statistical significance of the measurements was determined using the Student’s t -test, with a two-tailed non-paired comparison. Accession codes: The atomic coordinates and structure factors for the structure of CARMIL 1–668 have been deposited in the Protein Data Bank with accession code 4K17 . How to cite this article: Zwolak, A. et al . CARMIL leading edge localization depends on a non-canonical PH domain and dimerization. Nat. Commun. 4:2523 doi: 10.1038/ncomms3523 (2013).